Cobalt phosphate-modified barium-doped tantalum nitride nanorod photoanode with 1.5% solar energy conversion efficiency Spurred by the decreased availability of fossil fuels and global warming, the idea of converting solar energy into clean fuels has been widely recognized. Hydrogen produced by photoelectrochemical water splitting using sunlight could provide a carbon dioxide lean fuel as an alternative to fossil fuels. A major challenge in photoelectrochemical water splitting is to develop an efficient photoanode that can stably oxidize water into oxygen. Here we report an efficient and stable photoanode that couples an active barium-doped tantalum nitride nanostructure with a stable cobalt phosphate co-catalyst. The effect of barium doping on the photoelectrochemical activity of the photoanode is investigated. The photoanode yields a maximum solar energy conversion efficiency of 1.5%, which is more than three times higher than that of state-of-the-art single-photon photoanodes. Further, stoichiometric oxygen and hydrogen are stably produced on the photoanode and the counter electrode with Faraday efficiency of almost unity for 100 min. The globally ongoing solar fuel projects reflect the pressing need for producing fuels from sunlight so that solar energy can be stored and used whenever and wherever it is needed [1] , [2] , [3] . Photoelectrochemical (PEC) splitting of water into hydrogen and oxygen is a promising way to directly convert solar energy into fuel [4] , [5] , [6] , [7] . Among the proposed configurations for PEC cells [6] , the dual band gap PEC cell constructed by electrically connecting an n -type photoanode and a p -type photocathode in series is the most economical one that has the potential to realize the 10% solar-to-fuel conversion efficiency required for practical application. Constructing such a PEC cell requires both a photoanode and photocathode with high activity for water oxidation and reduction. Although many highly active and stable p -type photocathodes have been developed in recent years [8] , [9] , [10] , [11] , [12] , the more challenging task is to develop a photoanode that can stably oxidize water into oxygen under sunlight with high efficiency. The poor stability because of the strong oxidizing conditions and the low efficiency because of the high overpotential of four-electron water oxidation are the major challenges in designing the photoanode. To the best of our knowledge, the solar energy conversion efficiency of single-photon photoanodes reported so far are below 0.5% at best [13] , [14] , [15] , [16] , [17] . Thus, there is still much room for improvement in the activity of the photoanode to achieve high efficiency in an integrated dual band gap PEC cell. A PEC cell is a complex system, every aspect of which should be optimized to maximize device performance. For the photoanode part, the structure, material properties and co-catalyst modification are the three determining factors of its efficiency. The use of nanostructures is an effective way to improve the efficiency of the photoanode as it results in enhanced carrier collection, improved light absorption and surface area-enhanced charge transfer [18] . Choosing a visible-light-responsive semiconductor with energy band positions that favour water oxidation and reduction is also effective in improving the efficiency of the photoanode. The semiconductor material properties can be further improved by doping with appropriate impurities, a technique that is indispensable in the semiconductor industry. Modification of the photoanode with a suitable oxygen evolution co-catalyst is equally important as it improves the efficiency by lowering the overpotential and preventing photocorrosion. Recently, we reported a highly efficient photoanode made of a vertically aligned tantalum nitride (Ta 3 N 5 ) nanorod array modified with an iridium oxide co-catalyst [15] . The photoanode, owing to its nanorod structure and Ta 3 N 5 material properties, exhibited state-of-the-art efficiency at the time of reporting. Yet, the solar energy conversion efficiency of this photoanode was still below 0.5%. Unintentionally doped Ta 3 N 5 is an n -type semiconductor with a band gap of 2.1 eV, capable of absorbing a large portion of the solar radiation, up to a wavelength of ~590 nm. The energy bands of Ta 3 N 5 straddle the water redox potentials [19] , which is energetically more suitable for water splitting than most visible-light-responsive oxides (for example, Fe 2 O 3 (ref. 14 ), WO 3 (ref. 20 ) and BiVO 4 (ref. 21 )), having a conduction band too positive for H 2 evolution. Ta 3 N 5 has been widely used for both photocatalytic and PEC water splitting [22] , [23] , [24] , [25] , [26] , [27] , [28] . Various attempts have been made to increase the activity of Ta 3 N 5 by doping with foreign elements, mostly with group IA alkali metals [29] , [30] , [31] . The effectiveness of doping demonstrated with alkali metals is still limited. Here we demonstrate that the efficiency of the Ta 3 N 5 nanorod photoanode is greatly improved by doping the nanorods with barium (Ba) and modifying the surface with cobalt phosphate (Co-Pi) as an oxygen evolution co-catalyst. The Co-Pi-modified Ba-doped Ta 3 N 5 (hereinafter Co-Pi/Ba-Ta 3 N 5 ) nanorod photoanode yielded a solar energy conversion efficiency of 1.5%, representing a leap forward in improving the efficiency of photoanode for PEC water splitting. Structural and crystallographic properties Ba-Ta 3 N 5 nanorods were fabricated on a Ta foil by nitridation of Ba(NO 3 ) 2 -loaded Ta 2 O 5 nanorods grown by through-mask anodization. For comparison, undoped Ta 3 N 5 nanorods were fabricated by nitridation of Ta 2 O 5 nanorods cut from the same sample without loading Ba(NO 3 ) 2 . 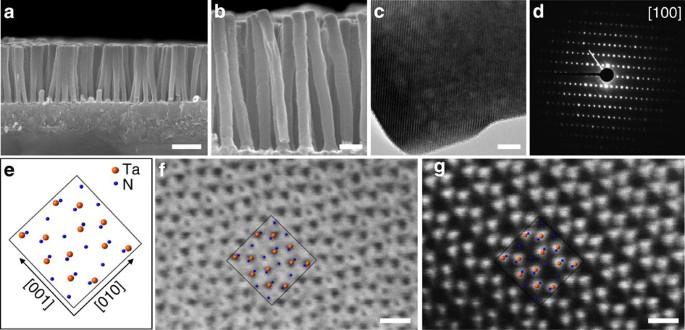Figure 1: Structural properties of the Ba-Ta3N5nanorods. (a,b) SEM images of the cross-section of the vertically aligned Ba-Ta3N5nanorod arrays. (c) High-resolution transmission electron microscopy image of a Ba-Ta3N5nanorod, taken along the [100] zone axis. (d) Corresponding selected area electron diffraction pattern acquired from the nanorod inc. (e) Crystal structure of Ba-Ta3N5viewed from the [100] crystallographic direction (from 3D-EDT data). (f) ABF and (g) HAADF scanning transmission electron microscopy images of a Ba-Ta3N5nanorod. Simulated cells of Ba-Ta3N5are overlaid infandg. Scale bars, (a) 300 nm, (b) 100 nm, (c) 10 nm, (f,g) 0.5 nm. Figure 1 shows the structural and crystallographic properties of the Ba-Ta 3 N 5 nanorods. The scanning electron microscopy (SEM) image in Fig. 1a reveals that the vertical alignment of the nanorods was retained after Ba doping. No obvious change in the morphology of the nanorods was found after Ba doping ( Supplementary Fig. S1 ). The diameter and length of the Ba-Ta 3 N 5 nanorods measured from the SEM image in Fig. 1b were ~60 and ~600 nm, respectively. Using highly sensitive energy dispersive X-ray spectroscopy (EDS), Ba signal was directly detected and the distribution of Ba on the surface of the sample was found to be uniform ( Supplementary Fig. S2 ). From the cross-sectional EDS mapping, it was found that Ba was incorporated not only on the surface of the sample but also into the sample ( Supplementary Fig. S3 ). The atomic concentration of Ba on the surface of the nanorods was estimated to be about 2.7% from X-ray photoelectron spectroscopy (XPS) spectra taken at a small take-off angle (20°; Supplementary Figs S4 and S5 ). An atomic concentration of 0.6% was estimated by EDS ( Supplementary Fig. S2 ). The difference between the XPS and EDS results suggests that the concentration of Ba on the surface may be higher than that in the bulk. The EDS and XPS results also revealed the existence of residual O in the nanorods. Using single crystal three-dimensional electron diffraction tomography (3D-EDT), both Ta 3 N 5 and Ba-Ta 3 N 5 nanorods have been found to have the same structure with space group symmetry Cmcm and unit cell parameters a =3.62 Å, b =10.04 Å, c =9.86 Å. The detailed structure solutions for Ta 3 N 5 and Ba-Ta 3 N 5 nanorods are given in Supplementary Figs S6–S9 and Supplementary Table S1 . At present, unfortunately 3D-EDT without dynamical scattering data corrections does not have enough sensitivity to detect substitutional probability of Ba for Ta and O for N. The high-resolution transmission electron microscopy image and the corresponding selected area electron diffraction pattern are shown in Fig. 1c,d . Both Ta 3 N 5 and Ba-Ta 3 N 5 nanorods reveal high single-crystalline quality with the structure mentioned above. Using scanning transmission electron microscopy with aberration corrector in probe, annular bright field (ABF) and high-angle annular dark field (HAADF) images of Ba-Ta 3 N 5 nanorods with atomic resolution were obtained. Figure 1e–g show, respectively, the obtained crystal structure of Ta 3 N 5 projected along the [100], and corresponding ABF and HAADF images. High crystallinity and the structural consistency were confirmed. The HAADF image clearly shows the distribution of heaviest Ta and Ba elements. Although there is a clear different between the atomic numbers of both elements, the low Ba concentration and its random distribution into the Ta positions prevent its direct visualization from the contrast of the HAADF image. The complementary information about the location of the light elements was obtained from the simultaneously recorded ABF image, where atomic columns of N and O randomly distributed are clearly observed. Figure 1: Structural properties of the Ba-Ta 3 N 5 nanorods. ( a , b ) SEM images of the cross-section of the vertically aligned Ba-Ta 3 N 5 nanorod arrays. ( c ) High-resolution transmission electron microscopy image of a Ba-Ta 3 N 5 nanorod, taken along the [100] zone axis. ( d ) Corresponding selected area electron diffraction pattern acquired from the nanorod in c . ( e ) Crystal structure of Ba-Ta 3 N 5 viewed from the [100] crystallographic direction (from 3D-EDT data). ( f ) ABF and ( g ) HAADF scanning transmission electron microscopy images of a Ba-Ta 3 N 5 nanorod. Simulated cells of Ba-Ta 3 N 5 are overlaid in f and g . Scale bars, ( a ) 300 nm, ( b ) 100 nm, ( c ) 10 nm, ( f , g ) 0.5 nm. Full size image In addition to changing the properties of the nanorods, the doping of Ba also drastically changed the properties of the interlayer between the nanorods and Ta substrate ( Fig. 1a ). This interlayer is grown simultaneously with the nanorods in the through-mask anodization process and its composition is a key factor affecting the activity of the nanorod photoanode. In our previous report [15] , we demonstrated that the interlayer was transformed into Ta 5 N 6 /Ta 2 N by using high-temperature nitridation, which enhanced the activity of the nanorod photoanode. The activity of the nanorod photoanode could be further improved if the less conductive Ta 5 N 6 phase is suppressed. It is therefore of particular interest to discover that the doping of Ba greatly suppressed the Ta 5 N 6 phase in the interlayer. As shown in Fig. 2 , the intensity of Ta 5 N 6 peaks in the X-ray diffraction (XRD) pattern of the Ba-doped sample was much reduced compared with that for the undoped sample. As a result, the conductivity of the Ba-doped interlayer, which mainly consisted of Ta 2 N, was enhanced by approximately three times compared with that of the undoped interlayer, which consisted of Ta 5 N 6 and Ta 2 N ( Supplementary Fig. S10 ). 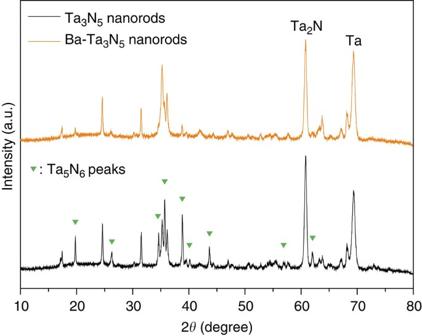Figure 2: XRD patterns for Ta3N5and Ba-Ta3N5nanorods. The diffraction peaks for the Ta5N6phase in the undoped sample are indicated by the green triangles. The Ta5N6phase in the interlayer was greatly suppressed by Ba doping. Figure 2: XRD patterns for Ta 3 N 5 and Ba-Ta 3 N 5 nanorods. The diffraction peaks for the Ta 5 N 6 phase in the undoped sample are indicated by the green triangles. The Ta 5 N 6 phase in the interlayer was greatly suppressed by Ba doping. Full size image Co-catalyst modification The coupling of an efficient light absorber with an active electrocatalysts is essential to make highly efficient photoelectrodes for water splitting. Especially for the photoanode, modifying the surface with an appropriate oxygen evolution electrocatalyst (co-catalyst) has an important role in lowering the overpotential and stabilizing the surface. The Co-Pi oxygen-evolving complex has, since its discovery [32] , raised wide interest in the water-splitting field, and has been used to modify various photoanodes to improve their activity and stability [20] , [21] , [33] , [34] , [35] , [36] . In our work, Co-Pi was employed as a co-catalyst for the Ba-Ta 3 N 5 nanorod photoanode. Without modifying Co-Pi, the nanorod photoanodes showed poor activity and stability ( Supplementary Fig. S11 ). The Co-Pi co-catalyst was deposited on the nanorod surface by photo-assisted electrodeposition in constant current mode at a small current density ( Supplementary Fig. S12 ). The deposition of Co-Pi under a small current density is believed to be beneficial to the formation of a uniform Co-Pi coating on the nanorods. The amount of the Co-Pi deposited on the surface of the sample was optimized to achieve both high activity and stability ( Supplementary Fig. S13 ). PEC water-splitting properties The PEC water-splitting properties of the Co-Pi/Ba-Ta 3 N 5 nanorod photoanode are given in Fig. 3 . The PEC properties of the Co-Pi/Ta 3 N 5 nanorod photoanode are also given for comparison. 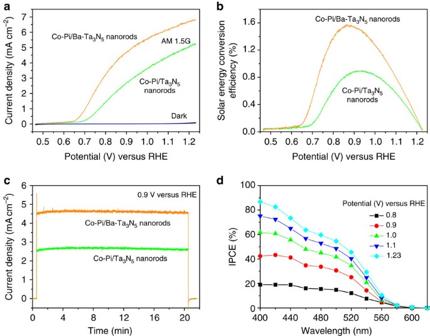Figure 3: Solar-driven PEC water-splitting properties. (a) Current–potential curves for Co-Pi/Ta3N5nanorod photoanode and Co-Pi/Ba-Ta3N5nanorod photoanode in dark and under AM 1.5G-simulated sunlight. (b) Solar energy conversion efficiency of the photoanodes calculated from the current–potential curves ina. (c) Steady-state photocurrent of the photoanodes held at 0.9 V versus RHE under AM 1.5G-simulated sunlight. (d) Wavelength dependence of IPCE for Co-Pi/Ba-Ta3N5nanorod photoanode at different applied potentials. Figure 3a shows the current–potential curves for the two electrodes in the dark and under air mass (AM) 1.5G-simulated sunlight. In the dark, both electrodes show negligible current. Under AM 1.5G, the photocurrent onset (measured at 0.2 mA cm −2 according to ref. 36 ) of the Ba-doped nanorod photoanode is at 0.65 V versus reversible hydrogen electrode (RHE), which shifts ~50 mV cathodically relative to the undoped sample. The sharp rise beyond the onset potential and the tendency for photocurrent saturation in the high-potential region indicate high-charge transfer and collection efficiency in the Co-Pi/Ba-Ta 3 N 5 nanorods. The photocurrent density of the Co-Pi/Ba-Ta 3 N 5 nanorod photoanode reaches 6.7 mA cm −2 at the water oxidation potential (1.23 V versus RHE). More importantly, high photocurrent density is achieved in the lower applied potential region. In the potential range of 0.7–1 V versus RHE, the photocurrent density in the Ba-doped sample is 1–5.5 mA cm −2 , which represents an increase of 50–300% compared with the undoped sample. Figure 3b plots the solar energy conversion efficiency of the two photoanodes calculated from the current–potential curves in Fig. 3a . The solar energy conversion efficiency is above 1% in the potential range of 0.75–1.05 V versus RHE for the Co-Pi/Ba-Ta 3 N 5 nanorod photoanode. A maximum conversion efficiency of 1.56% is achieved at 0.87 V versus RHE, as compared with the 0.89% at 0.93 V versus RHE for the undoped sample. It should be noted that the efficiency of the undoped Ta 3 N 5 nanorod photoanode is also much enhanced compared with our previous report (ref. 15 ) owing to the improved co-catalyst modification method. Nanorods with different diameters and densities have been tested, which showed that the nanorods used above gave the highest efficiency ( Supplementary Fig. S14 and Supplementary Table S2 ). Figure 3: Solar-driven PEC water-splitting properties. ( a ) Current–potential curves for Co-Pi/Ta 3 N 5 nanorod photoanode and Co-Pi/Ba-Ta 3 N 5 nanorod photoanode in dark and under AM 1.5G-simulated sunlight. ( b ) Solar energy conversion efficiency of the photoanodes calculated from the current–potential curves in a . ( c ) Steady-state photocurrent of the photoanodes held at 0.9 V versus RHE under AM 1.5G-simulated sunlight. ( d ) Wavelength dependence of IPCE for Co-Pi/Ba-Ta 3 N 5 nanorod photoanode at different applied potentials. Full size image Figure 3c shows the steady-state photocurrent of the photoanodes measured at 0.9 V versus RHE under AM 1.5G. It was found that the steady-state photocurrent densities were equal to the photocurrent densities of the current–potential curves in Fig. 3a , thus confirming that the conversion efficiency calculated from the current–potential curves represent steady-state behaviour. Both samples showed a stable photocurrent for 20 min, demonstrating that the Co-Pi co-catalyst modified using our method was effective in preventing self-oxidation of the Ta 3 N 5 and Ba-Ta 3 N 5 nanorods. Recently, there has been some debate about whether Co-Pi acts as a catalyst or spectator [36] , [37] , [38] . We believe that in our case the Co-Pi functions as a catalyst because otherwise self-oxidation would result if the water oxidation occurred on the Ta 3 N 5 or Ba-Ta 3 N 5 sites. Figure 3d plots the wavelength dependence of the incident photon-to-current conversion efficiency (IPCE) for the Co-Pi/Ba-Ta 3 N 5 nanorod photoanode measured at different applied potentials (see Supplementary Fig. S15 ). The Tauc plots of the IPCE spectra in Supplementary Fig. S16 reveals that the band gap of the Ba-Ta 3 N 5 nanorods is ~2.1 eV, same as that of undoped Ta 3 N 5 . At the water oxidation potential (that is, 1.23 V versus RHE, where the IPCEs of different photoanodes are usually compared), the IPCEs are 55–86% in the 500–400 nm range. Even at lower applied potentials, the IPCEs are quite high in this range. The relatively low IPCEs above 500 nm indicate the possibility of further improving the overall efficiency of the photoanode by enhancing the efficiencies in this region of spectrum. By integrating the IPCE spectrum measured at 1.23 V versus RHE in Fig. 3d over the spectrum of the AM 1.5G (ASTM G173-03), a photocurrent density of ~6.3 mA cm −2 was estimated, which was close to that of ~6.7 mA cm −2 measured from the current–potential curve in Fig. 3a ( Supplementary Fig. S17 ). This demonstrates that the current–potential curves measured using our solar simulator and the IPCE data are of good accuracy. To confirm that the reactions taking place on the Co-Pi/Ba-Ta 3 N 5 nanorod photoanode and the Pt counter electrode are the oxygen evolution reaction (OER) and hydrogen evolution reaction (HER), respectively, the gases evolved from both electrodes were quantified by gas chromatography ( Fig. 4 ). The Co-Pi/Ba-Ta 3 N 5 nanorod photoanode was held at 0.9 V versus RHE under AM 1.5G for 100 min. The amount of electrons passing through the outer circuit was 265 μmol cm −2 during the 100 min. The amounts of O 2 and H 2 evolved from the Co-Pi/Ba-Ta 3 N 5 nanorod photoanode and the Pt counter electrode were 63.5 and 130 μmol cm −2 , respectively. The ratio of evolved O 2 and H 2 is close to stoichiometry, and the Faraday efficiencies of the OER and HER are 96% and 98%, respectively. These results suggest that the photocurrent is indeed due to the OER and HER and the conversion efficiency calculated from the photocurrent does represent the solar-to-hydrogen conversion efficiency of the photoanode. The results also demonstrate that the photoanode has good stability for the OER. The photocurrent decayed by only 5% after 100 min ( Supplementary Fig. S18 ). 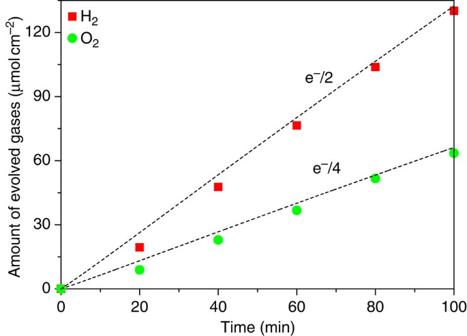Figure 4: Gas chromatography of the oxygen and hydrogen evolved from the electrodes. The photoanode was biased at 0.9 V versus RHE. The dashed lines indicate the expected amount of oxygen and hydrogen evolution with unity Faraday efficiency. Figure 4: Gas chromatography of the oxygen and hydrogen evolved from the electrodes. The photoanode was biased at 0.9 V versus RHE. The dashed lines indicate the expected amount of oxygen and hydrogen evolution with unity Faraday efficiency. Full size image To exclude the effect of nitrate ions (NO 3 − ) on enhancing the PEC activity of Ta 3 N 5 nanorods, different nitrate precursors including NaNO 3 , Mg(NO 3 ) 2 and Al(NO 3 ) 3 were used to treat the sample under the same process as that for the Ba(NO 3 ) 2 precursor. The concentrations of NO 3 − in the aqueous solutions were kept at 0.2 M for all nitrate precursors. As shown in Supplementary Fig. S19 , the suppression of Ta 5 N 6 phase was only found in the Ba(NO 3 ) 2 -treated sample. Compared with undoped sample in Fig. 3a , the NaNO 3 - and Mg(NO 3 ) 2 -treated samples showed even lower activity, whereas the Al(NO 3 ) 3 -treated sample showed only slightly enhanced activity, not comparable to the Ba(NO 3 ) 2 -treated sample. The effect of Ba doping on enhancing the PEC activity of the Ta 3 N 5 nanorods was further demonstrated by treating the sample with different Ba precursors. Aqueous solutions of Ba(NO 3 ) 2 , barium chloride and barium acetate with the same concentration (0.1 M) were used as Ba precursors to treat the samples under the same condition. As shown in Supplementary Fig. S20 , the suppression of Ta 5 N 6 phase was found in all the samples treated with these Ba precursors. All the samples showed similar PEC activity, which were much enhanced compared with that of the undoped sample in Fig. 3a . The above results excluded the effect of NO 3 − and confirmed the effect of Ba on enhancing the PEC activity of Ta 3 N 5 nanorods. The concentration of the Ba(NO 3 ) 2 precursor was also optimized, which was found to be 0.1 M ( Supplementary Fig. S21 ). The enhancing effect of Ba doping on PEC activity of the Ta 3 N 5 nanorod photoanode is ascribed to the enhanced electrical conductivity of the interlayer and the improved surface and bulk properties of the nanorods for water splitting. The enhanced conductivity of the interlayer was achieved by suppressing the Ta 5 N 6 phase in the interlayer, which allowed the electrons to be collected more efficiently at the back contact. The doping of Ba could improve the properties of the Ta 3 N 5 nanorods for water splitting in two aspects. First, the surface hydroxyl concentration of the nanorod is increased because Ba on the surface easily bonds with hydroxyl ions in the electrolyte. The adsorption of these potential-determining ions on the nanorod surface could change the interfacial energetics and shift the flatband potential [18] . Indeed, a Mott–Schottky analysis ( Supplementary Fig. S22 ) showed that the flatband potential of the Ba-Ta 3 N 5 nanorods shifted cathodically by 90 mV relative to that of the undoped Ta 3 N 5 nanorods. The cathodic shift of the flatband potential could contribute to the shift of the onset potential of the current-potential curves and improved PEC activity observed in Fig. 3a . A similar enhancing effect of Ba doping on the photocatalytic water-splitting activity of La 2 Ti 2 O 7 because of increased surface hydroxyl concentration has been reported [39] . The results suggest a way to improve the efficiency of the photoelectrode by controlling the potential-determining ions. Second, the carrier density in the nanorod was increased by >50% after doping with Ba ( Supplementary Fig. S22 ). The increased carrier density could lead to more efficient electron transfer in the nanorods. As a consequence of the synergistic effects of enhanced interlayer conductivity, cathodically shifted flatband potential, and increased electron density in the nanorods, the PEC activity of the Ta 3 N 5 nanorod photoanode was improved after Ba doping. In conclusion, we demonstrated an efficient and stable photoanode for water splitting by coupling an intentionally doped semiconductor nanostructure (that is, Ba-Ta 3 N 5 nanorod) with a stable OER co-catalyst (that is, Co-Pi). The Co-Pi/Ba-Ta 3 N 5 nanorod photoanode yielded a maximum solar energy conversion efficiency of 1.5%. To our knowledge, this is more than three times higher than the current state-of-the-art solar energy conversion efficiency of single-photon photoanodes for PEC water splitting. Further, stoichiometric O 2 and H 2 were stably produced on the Co-Pi/Ba-Ta 3 N 5 nanorod photoanode and the Pt counter electrode with Faraday efficiency of almost unity. This represents a leap forward in pursuing the 10% solar-to-fuel conversion efficiency goal and further efforts are being made to shift the photocurrent onset, boost the efficiency at longer wavelengths, as well as improve the long-term stability. Preparation of nanorod photoelectrodes Vertically aligned Ta 2 O 5 nanorods were grown on a Ta foil (0.1 mm in thickness, 1 × 5 cm 2 in size) by through-mask anodization. A Ta foil (99.95%, Nilaco) with a thickness of 0.1 mm was cut into 1 × 5 cm 2 pieces and cleaned in acetone and isopropyl alcohol. An Al layer with a thickness of ~2 μm was deposited on the Ta substrate by thermal evaporation. The Al layer was anodized in 0.3 M oxalic acid at 40 V for 2 h to form a porous anodic alumina (PAA) mask. Subsequently, the nanochannels of the PAA mask were widened by dipping into a 5% H 3 PO 4 aqueous solution at 60 °C for 90 s. The masked Ta substrates were then anodized in a 0.5-M H 3 BO 3 aqueous solution at room temperature under stirring. The anodizing voltage was ramped from 0 to 650 V at a rate of 0.1 V s −1 and held at 650 V for 1 h. The Ta 2 O 5 nanorods embedded into the PAA mask were released by selectively etching away the PAA mask with a 5% H 3 PO 4 aqueous solution at 60 °C for 4 h. The obtained Ta 2 O 5 nanorod array was further cut into 5 × 10 mm 2 pieces. The Ba precursor was introduced by dipping the Ta 2 O 5 nanorods into an aqueous solution of 0.1 M Ba(NO 3 ) 2 for ~10 s and dried with a N 2 gun. Ba-Ta 3 N 5 nanorods and Ta 3 N 5 nanorods were obtained by nitridation of Ta 2 O 5 nanorods with and without Ba in a horizontal tube furnace under 5 sccm NH 3 flow at 1,000 °C for 2 h. Electrical contact was established by embedding a Cu wire in a eutectic gallium–indium alloy (Aldrich) that contacted the bottom Ta layer of the sample. The Cu wire and the eutectic were covered with Kapton tape (Nitto Tape) and then encapsulated with epoxy (Araldite). The exposed area of the electrode after packaging was about 0.4 cm 2 . Photo-assisted electrodeposition of Co-Pi co-catalyst Before Co-Pi deposition, the electrode was immersed in a mixed etchant of HF:HNO 3 :H 2 O (1:2:7 in v/v) for 10 s and rinsed with pure water. The freshly prepared electrode was transferred to a three-electrode PEC cell for photo-assisted electrodeposition of the Co-Pi co-catalyst. The nanorod electrode was used as the working electrode, Ag/AgCl as the reference electrode and a Pt wire as the counter electrode. The Co-Pi cocatalyst was deposited in a stirred solution of 0.5 mM Co(NO 3 ) 2 in 0.1 M potassium phosphate buffer at pH 7 at a constant current density of 10 μA cm −2 over a period of 8 min under AM 1.5G-simulated sunlight. After deposition, the electrode was rinsed with pure water. Structural characterization SEM images of the nanorods were taken with a Hitachi S-4700 at an accelerating voltage of 20 kV. XRD patterns of the samples were measured with a Rigaku Ultima III using Cu K α radiation at 40 kV and 40 mA. XPS spectra were measured with a JEOL JPS-9010 using non-chromatic Al K α radiation at 12 kV and 25 mA. The electron analyser was operated at pass energies of 50 eV for wide scan and 10 eV for narrow scan, which gave full width at half maximum of 1.8 and 0.9 eV for the Ag 3d 5/2 peak, respectively. XPS spectra were measured at take-off angles of 90° and 20°. The peak shift due to charging was corrected using the C1s peak at 285 eV as an internal standard. Quantitative XPS analysis was done using a relative sensitivity factor method. High-resolution transmission electron microscopy images, selected area electron diffraction patterns and 3D-EDT were recorded on a JEOL 2100 (LaB 6 filament) with Cs=1.4 mm operated at 200 kV. Samples were prepared by scratching nanorods on a filter paper using tweezers, and then a copper grid was put on to stick some nanorods. After that, the TEM grid was heated for 2 h under lamp. Diffraction patterns in 3D reciprocal space were collected in accessible angular range by combination of electron-beam tilt and sample-holder tilt with a designated step. Herein the total range of angles covered for both samples are over 120° with 0.1 × step. HAADF and ABF scanning transmission electron microscopy images were acquired with a JEOL JEM-ARM200F equipped with a Cs-aberration corrector in condenser lens operated at 200 kV provided with a spherical aberration corrector in probe (current emission density ~1.4 × 10 −9 A and probe size ~0.8 A), a GIF-QuantumER spectrometer and Oxford INCA-350 detector. Solid semiangles between 68–280 mrad and 11–22 mrad were used for acquisition of HAADF and ABF images, respectively (38 s per frame). EDS spectra and elemental maps were taken with a JEOL JSM-7800F equipped with a highly sensitive silicon drift detector (Oxford Instruments, X-Max N 150) at an effective solid angle of 0.042 sr and an accelerating voltage of 8 kV. PEC measurements PEC water-splitting properties of the nanorod photoelectrodes were measured with the three-electrode configuration using an Ag/AgCl reference electrode and a Pt wire counter electrode. The potential of the working electrode was controlled by a potentiostat (Hokuto Denko, HSV-100). The measured potential versus Ag/AgCl was converted to the RHE scale according to the Nernst equation ( E RHE =E Ag/AgCl +0.059 pH+0.197). An aqueous solution of 0.5 M K 2 HPO 4 was used as the electrolyte. The pH of the electrolyte was adjusted to 13 by adding KOH. The electrolyte was stirred and purged with Ar gas before the measurements. The photoelectrodes were illuminated with AM 1.5G-simulated sunlight at 100 mW cm −2 from a commercial solar simulator (SAN-EI Electric, XES-301 S). Current–potential curves were measured at a scan rate of 10 mV s −1 from negative to positive. Solar energy conversion efficiency ( η ) of the photoanode (defined in ref. 6 for an individual photoelectrode) was calculated from the current–potential curves measured in the dark and under AM 1.5 G with the equation η= [1.23− V app ) × ( J light − J dark )/ P light ] × 100%, where V app is the applied potential versus RHE, J dark and J light are the respective current densities in the dark and under AM 1.5 G and P light is the power density of AM 1.5G (100 mW cm −2 ). The wavelength dependence of IPCE was measured under monochromatic irradiation from a Xe lamp (Asahi Spectra, MAX-302) equipped with bandpass filters (central wavelengths: 400–620 nm, every 20 nm; full width at half maximum: 10 nm). The irradiance spectra of the light incident on the electrode surface were measured with a spectroradiometer (EKO Instruments, LS-100). The IPCE at each wavelength ( λ ) was calculated via the equation IPCE=[(1240/ λ ) × ( J light − J dark )/ P light ] × 100%. Gas chromatography An air-tight three-electrode PEC cell with an Ag/AgCl reference electrode and a Pt wire counter electrode was used for gas chromatography. The PEC cell was connected to a vacuum pump and a gas chromatograph. Before measurement, the PEC cell was pumped to a base pressure of a few Torr (because of the vapour pressure of water) and then backfilled with Ar to about 40 Torr. The Co-Pi/Ba-Ta 3 N 5 nanorod photoelectrode was biased at 0.9 V versus RHE in a stirred aqueous solution of 0.5 M K 2 HPO 4 (pH=13) under AM 1.5G-simulated sunlight. The amount of oxygen and hydrogen evolved from the photoelectrode and the Pt counter electrode were measured with a gas chromatograph (Shimadzu, GC-8A). How to cite this article: Li, Y. et al. Cobalt phosphate-modified barium-doped tantalum nitride nanorod photoanode with 1.5% solar energy conversion efficiency. Nat. Commun. 4:2566 doi: 10.1038/ncomms3566 (2013).